Low-temperature carbon monoxide oxidation catalysed by regenerable atomically dispersed palladium on alumina Catalysis by single isolated atoms of precious metals has attracted much recent interest, as it promises the ultimate in atom efficiency. Most previous reports are on reducible oxide supports. Here we show that isolated palladium atoms can be catalytically active on industrially relevant γ-alumina supports. The addition of lanthanum oxide to the alumina, long known for its ability to improve alumina stability, is found to also help in the stabilization of isolated palladium atoms. Aberration-corrected scanning transmission electron microscopy and operando X-ray absorption spectroscopy confirm the presence of intermingled palladium and lanthanum on the γ-alumina surface. Carbon monoxide oxidation reactivity measurements show onset of catalytic activity at 40 °C. The catalyst activity can be regenerated by oxidation at 700 °C in air. The high-temperature stability and regenerability of these ionic palladium species make this catalyst system of potential interest for low-temperature exhaust treatment catalysts. Automotive catalytic converters have played a central role in improving air quality in urban environments. Platinum group metals constitute the catalytically active phase that helps to mitigate pollutants such as hydrocarbons, nitrogen oxides and CO, thus helping reduce smog and ozone. Exhaust treatment catalysts are very effective when heated above 200 °C, but provide limited reactivity at lower temperatures because these metals are poisoned by CO at lower temperatures. As a consequence, most of the pollutants from a modern automobile are emitted during the first 30 s of starting a car, when the catalyst is still being warmed up. There is a need to develop catalysts that are not poisoned by CO and become active at low temperatures. The US Department of Energy road map has set a goal for light-off below 150 °C (ref. 1 ). Herein we demonstrate that atomically dispersed Pd 2+ ions, bound to surface oxygen atoms on alumina, resist CO poisoning and are able to achieve high activity for CO oxidation at low temperatures. A recent report by Flytzani-Stephanopoulos [2] reviews the evidence that atomically dispersed, ionic Au species are present on Au/TiO 2 and are responsible for increased catalytic reactivity. Similar results on single-atom catalysts were reported by for Pt on the reducible oxide FeO x (ref. 3 ). There is increasing interest in catalysis by single atoms, which promise high atom efficiency and improved low-temperature reactivity, as well as selectivity. For example, Ir/FeO x (ref. 4 ) and Pd/CeO 2 (ref. 5 ) also exhibit improved low-temperature reactivity, which may be related to the presence of atomically dispersed species. However, in each of these catalysts, the support is a reducible metal oxide that can provide labile oxygen species that can participate in the reaction. In our work we have focused on γ-alumina as a support, as it is the most widely commercialized support for heterogeneous catalysts due to its high specific surface area (100–200 m 2 g −1 ) and thermal stability. The structure of γ-alumina can be thought of as an fcc (face centred cubic) packing of oxygen atoms, with Al 3+ cations filling octahedral and tetrahedral interstitial sites among the oxygen atoms. The γ-alumina structure has been considered as a defective spinel structure [6] , in which the Mg 2+ atoms in spinel (MgAl 2 O 4 ) have been removed and the Al 2 O 3 stoichiometry is accommodated by cation vacancies. More recently, a non-spinel structure, energetically more stable and more reflective, of experimental data has been proposed [7] , [8] . This structural model also has the advantage of being practical for density functional theory (DFT) calculations, capturing the essence of the γ-alumina structure in a smaller unit cell than the spinel structure, and is the model used in our work. For consistency with the literature, however, Miller indices used in this work refer to the spinel unit cell. Both the defective spinel and the non-spinel models proposed for the γ-alumina structure contain Al 3+ vacancy-defect sites, manifested as four-fold hollow sites on the γ-alumina (100) surface. A second feature, common to all models, are penta-coordinated Al 3+ surface sites, also known as coordinatively unsaturated Al 3+ sites [9] , [10] , formed by the truncation of AlO 6 octahedra at the γ-alumina (100) surface. In practice, high working temperatures inevitably lead to the transformation of the transitional γ-alumina to thermodynamically stable corundum, with concomitant loss of surface area. However, the addition of a few mol% La 2 O 3 to γ-alumina has been found to result in improved surface area stability at high temperatures [11] , [12] , [13] . Using X-ray photoelectron spectroscopy (XPS), Haack et al . [14] determined that for La/Al ratios <0.15, La is probably present as a dispersed, low-coordinated La 3+ phase, rather than as La 2 O 3 . Lanthanum oxide has been routinely added to γ-alumina in automobile catalysts since these discoveries, but the location of the La 3+ was somewhat of a mystery until the advent of aberration-corrected (AC) electron microscopes, in conjunction with DFT calculations. It was shown by Wang et al . [15] that atomically dispersed La 3+ is present on the γ-alumina surface, settling into four-fold hollow, Al 3+ vacancy sites. These surface La 3+ ions appear to pin the oxygen substructure, hindering the reconstructive transformation from the fcc (abcabc…) arrangement to the hcp (hexagonally close packed) (ababab…) packing of the corundum structure. In the case of palladium, XPS observations by Otto et al . [16] demonstrated the existence of two types of palladium oxide present on γ-alumina. One oxide was characterized by relatively large particles with a Pd 3 d binding energy characteristic of PdO, and which could be readily transformed to Pd metal at room temperature in hydrogen. The second oxide, predominant at low palladium loadings (≤0.5 wt%), was characterized by a binding energy shift of 1.6 eV, higher than that for PdO, and was found to be resistant to reduction to Pd metal at room temperature in hydrogen. It was proposed by these authors that this second chemical state of palladium could correspond to highly dispersed Pd 2+ due to a strong metal–support interaction. More recently, palladium has been observed to be stabilized as an atomically dispersed, as well as catalytically active species, on mesoporous alumina [17] . At low Pd loadings (<0.1 wt%), the Pd present on this support was observed to be predominantly atomically dispersed as Pd 2+ . It was also found that these species were catalytically active for the selective aerobic oxidation of allylic alcohols. There are, however, no reports of the stabilization of atomically dispersed Pd at elevated temperatures, such as those encountered in automotive catalysts. This work has focused on the synergistic effects of La and Pd, supported on γ-alumina. We compare the CO oxidation reactivity of atomically dispersed Pd, loaded onto pure γ-alumina and La-doped γ-alumina supports. Aberration-corrected electron microscopy was used to characterize dispersion of La and Pd species on the surface of the γ-alumina support. To correlate catalytic behaviour with the chemical state of Pd, simultaneous CO oxidation and Pd K-edge X-ray absorption spectroscopy (XAS) measurements were also performed. On the basis of these experiments, coupled with DFT calculations, a structural model for atomically dispersed Pd on La-alumina is proposed, as well as a possible CO oxidation mechanism. Imaging of atomically dispersed Pd In previous work [18] , we reported the role of lanthana on the particle size of Pd and the reactivity for CO oxidation in a 2.5 wt% Pd/Al 2 O 3 catalyst. At this high metal loading, most of the Pd is present in the form of metallic nanoparticles. However, we noticed that Pd particles on the La-alumina support were smaller, were more readily oxidized and desorbed CO at low temperatures, mitigating the poisoning effect. As a result, there was a modest improvement in low-temperature performance of the Pd/La-alumina catalysts, compared with the Pd/alumina. In addition, high-angle annular dark-field transmission electron microscopy (HAADF TEM) coupled with energy-dispersive X-ray spectroscopy (EDS) provided evidence for the presence of atomically dispersed Pd and La in this catalyst. 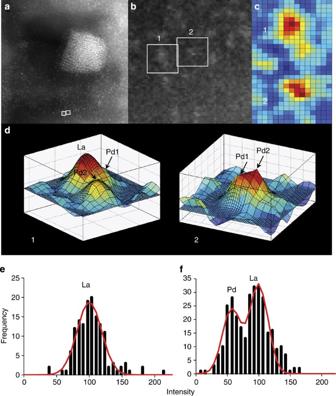Figure 1: Intensity analysis of Aberration Corrected Electron Microscope images. The images were obtained from a La-stabilized γ-alumina support sample with a 2.5 wt% Pd loading. (a) A typical region of the sample, with a Pd-metal particle surrounded by atomically dispersed Pd and La. (b) An enlarged region froma, showing two regions containing atomically dispersed species. (c) Colourized intensity maps from regions 1 and 2. (d) Two-dimensional (2D) Gaussian-function fits (fine-mesh) to the intensity maps inc. (e,f) Normalized intensity distributions, obtained from 2D Gaussian-function fits of images obtained from La-alumina (e) and Pd-La-alumina (f) showing well-resolved peaks corresponding to Pd and La electron backscatter intensity in the case of the Pd-La-alumina sample. The red lines represent Gaussian-function least-squares fits to the intensity distributions. Supplementary Figure 1 shows an EDS spectrum of a region of this 2.5 wt% Pd catalyst that is devoid of Pd-metal particles. Both Pd and La characteristic X-ray peaks are seen in the spectrum, indicating that these elements are present on the γ-alumina support at concentrations high enough to be detected by EDS but otherwise not visible in the HAADF images. The average concentration of the atomically dispersed Pd was estimated to be ~0.5 wt% and this loading is similar to that seen previously in automotive catalysts for the ‘oxidized’ form of Pd, which was thought to interact strongly with the alumina support [16] . An image of the 2.5 wt% Pd/La-alumina catalyst, obtained using an AC microscope is shown in Fig. 1a . This image confirms that isolated single atoms (the bright dots) are present on the alumina support in close proximity to the Pd metal nanoparticle. The contrast of these isolated single atoms results from electron scattering from the nucleus, with intensity related approximately to the square of the atomic number ( Z 2 ). The dependence of contrast on atomic number has previously been employed to distinguish the identity of individual atoms in a thin sample of boron nitride [19] , but application of this approach to identify the single atoms in a heterogeneous catalyst is more difficult due to the strong and varying background from the alumina support. We developed a method of image analysis that involves fitting the overlapping atom intensities to two-dimensional Gaussian functions ( Fig. 1b–d ), allowing for the extraction of single-atom intensities and facile background subtraction. The histogram of intensities shows a bimodal distribution for Pd/La-alumina ( Fig. 1f ), while a single peak is seen for the La-alumina sample (no Pd) ( Fig. 1e ). The ratio of image intensities (that is, peak positions on the x axis) of the two peaks in the bimodal distribution agrees with the ratio of the square of the atomic numbers for La and Pd, indicating that the atomically dispersed species, seen in Fig. 1a , are composed of Pd that is comingled with La on the alumina support. Figure 1: Intensity analysis of Aberration Corrected Electron Microscope images. The images were obtained from a La-stabilized γ-alumina support sample with a 2.5 wt% Pd loading. ( a ) A typical region of the sample, with a Pd-metal particle surrounded by atomically dispersed Pd and La. ( b ) An enlarged region from a , showing two regions containing atomically dispersed species. ( c ) Colourized intensity maps from regions 1 and 2. ( d ) Two-dimensional (2D) Gaussian-function fits (fine-mesh) to the intensity maps in c . ( e , f ) Normalized intensity distributions, obtained from 2D Gaussian-function fits of images obtained from La-alumina ( e ) and Pd-La-alumina ( f ) showing well-resolved peaks corresponding to Pd and La electron backscatter intensity in the case of the Pd-La-alumina sample. The red lines represent Gaussian-function least-squares fits to the intensity distributions. Full size image As the concentration of the atomically dispersed species in the 2.5 wt% Pd catalyst was estimated to be 0.5 wt%, we prepared a series of catalysts with this lower loading. The rest of the manuscript describes the characteristics of these 0.5 wt% Pd/alumina catalysts. An AC-scanning TEM (STEM) image of this catalyst is shown in Supplementary Fig. 2 . Bright dots corresponding to atoms of Pd and La are seen. The number of these bright dots were counted and when normalized to the surface area, the concentration was found to be consistent with the loading of this sample, as explained in the Supplementary Discussion . Hence, we conclude that when prepared carefully and calcined in air, these catalysts do not show any particulate Pd phase as seen by XRD, TEM or extended X-ray absorption fine structure (EXAFS). When studying the reactivity of atomically dispersed Pd species, it is important to prepare samples devoid of metallic Pd particles so that the reactivity can be ascribed to only one form of Pd. In previous work with Au catalysts, the authors had to leach out the metallic component before performing catalytic tests [2] , [20] . Even if the initial catalyst is in the form of atomically dispersed species, the catalyst can evolve during reaction measurement, as shown by Guan et al . [21] and, more recently, by Corma et al . [22] These authors suggest that atomically dispersed species can serve as precursors for the formation of very small clusters of the metal. Hence, it is necessary to use in situ spectroscopy to confirm the identity of the species responsible for catalytic reactivity. In this work we used XAS while performing reaction rate measurements to confirm the role of atomically dispersed Pd for low temperature CO oxidation. CO oxidation reactivity To probe the catalytic behaviour of these samples, we used the CO oxidation reaction under conditions of a modest excess of O 2 (~50% excess O 2 ). For metallic Pd under these conditions, CO oxidation is known to be positive first order with respect to O 2 , and negative first order with respect to CO [23] . The negative first-order kinetics for CO oxidation on platinum group metals are caused by the inhibition due to strong binding of CO to the metal surface. CO acts as a poison and must desorb before the reaction can proceed. When CO is removed from the surface, the catalyst ‘lights-off’ with the rate increasing quickly with increasing reaction temperature. The exothermic reaction makes the process autocatalytic, allowing 100% conversion to be achieved rapidly. Although light-off curves are useful for benchmarking catalyst performance, to derive kinetics we need to perform measurements at low conversion. We first describe the light-off characteristics of these catalysts and then explore the reaction kinetics. The light-off curves ( Fig. 2 ) were obtained by monitoring CO 2 formation as the catalyst was ramped from room temperature to 300 °C at a rate of 2 °C min −1 . The catalyst was then cooled to room temperature in the reaction mixture and a second light-off was performed to investigate the stability of the atomically dispersed Pd 2+ species. As can be seen in Fig. 2 , the first light-off curve for the Pd/La-alumina catalyst shows a distinct S-shape with a positive curvature (negative second derivative) at high conversions during the first cycle. The second light-off curve shows a similar shape as the first one, but as higher conversions are approached, we see a second inflexion point as the curve changes to a negative curvature (positive second derivative). In contrast to the light-off curves for Pd/La-alumina, the Pd/alumina catalyst shows only a sharp increase in CO oxidation reactivity as higher conversions are reached (negative curvature). These characteristic shapes of the light-off curves are indicative of a shift in reaction order for CO oxidation from positive order in the case of the S-shaped curve to a negative order for the curves that rise sharply at higher conversions [24] . A negative order of reaction leads to an increase in reaction rate as adsorbed CO is depleted at high conversions. As metallic Pd shows a negative order of reaction with respect to CO, the observed changes in the light-off curves suggest that the Pd 2+ is being reduced during reaction, forming metallic Pd. 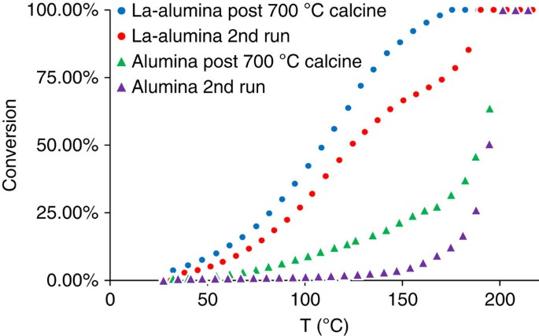Figure 2: CO-oxidation light-off curves for 0.5 wt% Pd on alumina and La-alumina. The first run was performed after calcining the sample,in situ, at 700 °C for 30 min. After the completion of the first run (Tmax=300 °C), the sample was cooled to room temperature in the reaction mixture and the second run was performed. Figure 2: CO-oxidation light-off curves for 0.5 wt% Pd on alumina and La-alumina. The first run was performed after calcining the sample, in situ , at 700 °C for 30 min. After the completion of the first run ( T max =300 °C), the sample was cooled to room temperature in the reaction mixture and the second run was performed. Full size image The deactivation of the catalyst was studied under isothermal conditions (70 °C) to investigate the stability of the high-activity state of these catalysts ( Supplementary Fig. 3 ) and we see that although the Pd/La-alumina and Pd/alumina deactivate at similar rates, the Pd/alumina sample reactivity eventually approaches 0 at 70 °C, while the Pd/La-alumina sample remains active. These longer-term isothermal reaction runs also confirm that the CO 2 formation is catalytic and not caused by the stoichiometric reduction of PdO to Pd, which would take <10 s at the flow rates we have used. The turnover frequencies (TOF) for CO oxidation were estimated assuming that all of the Pd was atomically dispersed; we find the TOF on Pd/La-alumina to be an order of magnitude greater than on metallic Pd with an activation energy of ~37 kJ mol −1 , considerably lower than the activation energy of 60–80 kJ mol −1 for metallic Pd ( Table 1 gives more details). The temperature dependence of the TOFs for Pd alumina, La-alumina and a reference sample of Pd metal powder are presented in Supplementary Fig. 4 . We also present analysis of transport effects under our experimental conditions and conclude that due to the low loading of Pd, the kinetic data at low conversion are not subject to any heat and mass transfer limitations (see Supplementary Discussion ). Table 1 Turnover frequencies and activation energies. * Full size table CO oxidation reaction kinetics Additional experiments were performed where the temperature was kept constant so that the reactivity as a function of reactant composition could be studied. As the sample reactivity was continuously decaying, the reaction orders were determined by switching reactant flows and comparing the changes in reaction rate before and after the switch in reactant flow rates ( Fig. 3 ). More details are provided in Supplementary Figs 5–8 and Supplementary Tables 2–5 , showing how the orders of reaction were derived. Even though the catalyst activity declines, the reaction order for the Pd/La-alumina sample is stable, with the CO reaction order remaining at +0.35 and the O 2 reaction order at +0.15 ( Table 2 ). The positive reaction order with respect to CO, seen for the Pd/La alumina is indicative of a reaction mechanism that is different from that seen on metallic Pd. It is clear that the presence of La helps to stabilize the chemical configuration responsible for the high reactivity of Pd 2+ for CO oxidation. The low positive order with respect to O 2 is consistent with a Mars van Krevelen mechanism, with the oxygen being derived from the surface, rather than the gas phase. 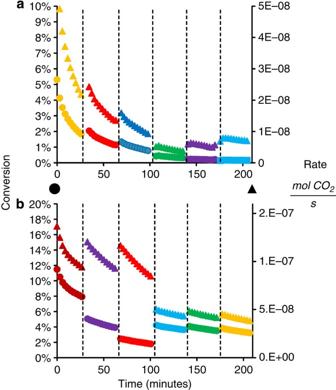Figure 3: Isothermal reaction rate measurements. Isothermal reaction rate measurements to determine orders of reaction for 0.5 wt% Pd on alumina (a) and on La-alumina (b). The reaction order for each reactant gas was obtained from the rate change occurring when one of the gas flows was increased or decreased. The circles refer to the left ordinate axis (% CO conversion) while the triangles refer to the right ordinate axis (rate—moles of CO2/s for 100 mg of catalyst). Figure 3: Isothermal reaction rate measurements. Isothermal reaction rate measurements to determine orders of reaction for 0.5 wt% Pd on alumina ( a ) and on La-alumina ( b ). The reaction order for each reactant gas was obtained from the rate change occurring when one of the gas flows was increased or decreased. The circles refer to the left ordinate axis (% CO conversion) while the triangles refer to the right ordinate axis (rate—moles of CO 2 /s for 100 mg of catalyst). Full size image Table 2 Reaction order with respect to CO and O 2 . * Full size table The Pd/alumina sample shows distinctly different behaviour. The reaction order for CO is negative (−0.2) and continues to decline with time on stream. The order of reaction with O 2 is +0.16 similar to that on Pd/La-alumina. A notable feature of this catalyst is a spike in CO 2 production for the first data point obtained while increasing the O 2 flow rate ( Supplementary Fig. 6 ). This spike suggests that metallic Pd is being oxidized and then this oxide gets converted to CO 2 as steady flows are established. Such spikes were not seen on the Pd/La-alumina catalyst. After the Pd/alumina has deactivated, it can be regenerated by oxidation at 700 °C and fresh catalyst reactivity behaviour is reproduced ( Supplementary Figs 6 and 7 ). However, if the catalyst is allowed to deactivate and not re-oxidized, the reaction kinetics change to approximately −1 order in CO and +1 order in O 2 , the behaviour expected for metallic Pd ( Supplementary Fig. 8 ). This is consistent with the change in reaction mechanism seen qualitatively by the changes in curvature in Fig. 2 , transitioning from a more reactive initial state and finally reverting to the behaviour of metallic Pd. The results suggest that although atomically dispersed Pd can be generated on alumina, these species are not stable and transform into a metallic phase. However, on La-alumina these species are more stable, as we show via operando XAS, discussed in the next section. Our reaction rate measurements were performed at temperatures up to 300 °C. Under these conditions, the loss of activity due to transformation to metallic Pd clusters was recovered fully via calcination in air. Operando X-ray absorption spectroscopy We examined the nature of the Pd during CO oxidation reaction via operando XAS at the Pd K-edge. For the operando study, reaction gases were passed through a vertical packed bed reactor positioned in the X-ray beam with exit gas compositions being analysed using a gas chromatograph. 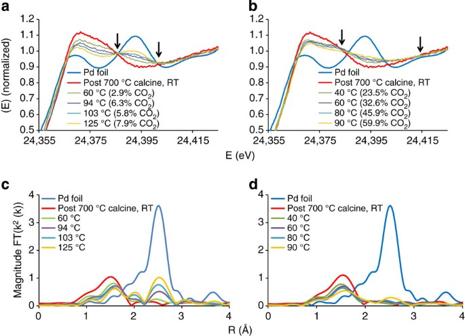Figure 4: XANES spectra and EXAFSk2-weighted Fourier transforms. Data were collected at multiple temperatures during CO oxidation, from samples composed of 0.5 wt% Pd on alumina (a,c) and on La-alumina (b,d). Arrows point to isosbestic points. Numbers in parentheses are the percent conversion of CO to CO2at the time of data collection. Figure 4 shows X-ray absorption near edge structure (XANES) and EXAFS data collected during CO oxidation over a range of temperatures (fits of the EXAFS data are shown in Supplementary Fig. 9 ). Isosbestic points, indicating that the spectra can be derived by a linear combination of two end member states, are marked by arrows in Fig. 4a,b . In Fig. 4a , it can be seen that the spectrum from the reference Pd foil passes through the isosbestic points shared by the 0.5 wt% Pd/alumina sample. This indicates that the spectra collected during CO oxidation can be represented by a linear combination of end member spectra collected from the initial, oxidized sample and from the foil. In contrast, as can be seen in Fig. 4b , it is apparent that the Pd foil reference spectrum does not pass through the isosbestic points formed by the spectra collected from the 0.5 wt% Pd/La-alumina sample in its initial state and during CO oxidation. For this sample, the spectra can be described as a linear combination of the initial state spectrum and a third chemical state for the Pd in this sample. This is also reflected in the EXAFS data ( Fig. 4c,d ). In the initial, oxidized state, both samples show only the peak associated with the Pd-O first shell. The absence of a second shell is evidence that in their initial state, neither sample contains any bulk PdO. In the case of the 0.5 wt% Pd/alumina sample, the decrease in the Pd-O first-shell peak height during CO oxidation is immediately accompanied by an increase in the Pd-metal first-shell peak height, reflecting the growth of Pd-metal at the expense of Pd-oxide. However, for the 0.5 wt% Pd/La-alumina sample, the PdO first-shell peak decreases immediately during CO oxidation at 40 °C, but no Pd-metal first-shell peak is seen until 90 °C. This is evidence for the presence of a third chemical state for Pd in this sample, characterized by an average Pd-O coordination that is significantly <4. The edge energy observed for this state (24,351.6±0.3 eV) falls between that for Pd metal (24,350 eV) and PdO (24,353 eV). The value of the edge energy for the active state, after accounting for experimental error, is sufficiently different from the Pd 0 and Pd 2+ reference compounds, indicating that this third chemical state is Pd 1+ . Figure 4: XANES spectra and EXAFS k 2 -weighted Fourier transforms. Data were collected at multiple temperatures during CO oxidation, from samples composed of 0.5 wt% Pd on alumina ( a , c ) and on La-alumina ( b , d ). Arrows point to isosbestic points. Numbers in parentheses are the percent conversion of CO to CO 2 at the time of data collection. 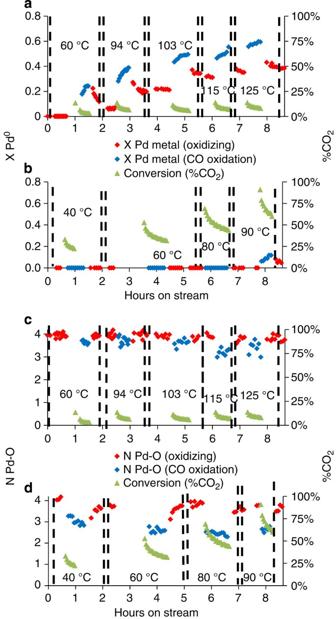Figure 5: Operando CO oxidation reaction/XAS measurements. Pd-metal fraction and CO conversion variation as a function of time and temperature during alternating CO oxidation reaction and oxidizing conditions. Pd loading 0.5 wt%. (a) Alumina support. (b) La-alumina support. (Pd-O coordination number and CO conversion variation as a function of time and temperature during alternating CO oxidation reaction and oxidizing conditions. (c) Alumina support. (d) La-alumina support. Full size image Figure 5 shows the time-resolved variations of the Pd-metal fraction (from linear combination fits of the XANES spectra) and the average Pd-O coordination number (from EXAFS data fits), respectively, together with the % CO conversion (from measurement of the CO 2 fraction in the exit gas). Gas compositions were switched between oxidizing conditions and CO oxidation by keeping the O 2 /He flowing and switching the CO flow on and off. This allowed any reduced Pd to become oxidized before restarting CO oxidation at the next higher temperature. In the case of the 0.5 wt% Pd/alumina sample, growth of Pd-metal is seen to begin immediately on exposure of the sample to CO oxidation conditions at 60 °C (blue), and the catalyst is seen to deactivate as the Pd-metal fraction increases ( Fig. 5a ). Partial recovery of the oxide species is obtained on switching to oxidizing conditions (red). The maximum CO conversion for this sample was ~13%. In contrast, the 0.5 wt% Pd/La-alumina sample shows no Pd-metal growth during CO oxidation until 90 °C, and again shows partial oxide species recovery on switching to oxidizing conditions ( Fig. 5b ). However, CO conversion is significantly higher for this sample, starting at ~20% at 40 °C and reaching close to 100% at 90 °C. Figure 5: Operando CO oxidation reaction/XAS measurements. Pd-metal fraction and CO conversion variation as a function of time and temperature during alternating CO oxidation reaction and oxidizing conditions. Pd loading 0.5 wt%. ( a ) Alumina support. ( b ) La-alumina support. (Pd-O coordination number and CO conversion variation as a function of time and temperature during alternating CO oxidation reaction and oxidizing conditions. ( c ) Alumina support. ( d ) La-alumina support. Full size image The EXAFS fitting procedure assumes that a separate Pd metal and oxide phase exists in the sample, the relative amounts determined from the XANES linear combination fits. Using the metal and oxide fractions, the coordination numbers were derived. The Pd-O first-shell coordination number for the 0.5 wt% Pd/alumina sample ( Fig. 5c ) is seen to decrease slightly from 4 during CO oxidation and fully recover on switching to oxidizing conditions. In contrast, for the 0.5 wt% Pd/La-alumina sample, the Pd-O coordination drops sharply to ~3 on exposure to CO oxidation conditions, recovering nearly fully when switching to oxidizing conditions ( Fig. 5d ). From this data, it is apparent that the presence of La in the Pd/γ-alumina catalyst stabilizes a state that is highly active towards CO oxidation. It was found that although the Pd/La-alumina catalyst deactivated with time on stream, it was possible to restore this catalyst to its initial state via a high-temperature oxidation treatment. 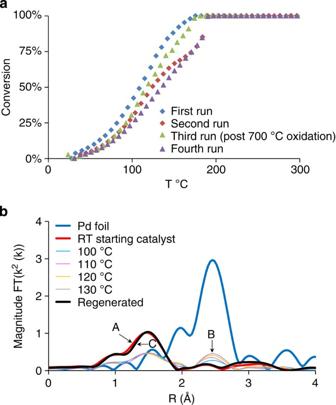Figure 6: Catalyst regeneration. (a) CO oxidation light-off curves for the 0.5 wt% Pd on La-alumina sample, showing that the catalyst is nearly regenerated after a 30 m, 700 °C oxidation treatment. (b) EXAFS Fourier transform plots showing (A) the state of the starting catalyst, and (B) the growth of Pd metal during CO oxidation. The catalyst was heated to 300 °C under CO oxidation and then re-oxidized at 700 °C, restoring the catalyst to its starting state (C). Figure 6a shows sequential light-off curves, obtained from the same Pd/La-alumina catalyst sample. The first run light-off curve shows the initial, high-activity state of the sample, while the second run curve displays partial deactivation. The sample was then treated, in place, to a 30 min, 700 °C oxidation treatment (1% O 2 /He). It can be seen by the third cycle that that the oxidation treatment has nearly restored the catalyst to its initial state. The fourth cycle again shows partial deactivation of the catalyst. Figure 6b (EXAFS Fourier transforms) shows the evolution of the Pd/La-alumina catalyst from its initial state, through CO oxidation at increasing temperatures, and finally to the restored state, following a 700 °C oxidation treatment. The initial state shows the Pd oxide first shell (Pd-O), with no Pd oxide second shell (Pd-Pd), which is indicative of atomically dispersed Pd (A). As CO oxidation occurs at increasing temperatures, the Pd metal first shell begins to grow in (B). The sample was taken to 300 °C under CO oxidation, and then to 700 °C in 1% O 2 /He. Figure 6: Catalyst regeneration. ( a ) CO oxidation light-off curves for the 0.5 wt% Pd on La-alumina sample, showing that the catalyst is nearly regenerated after a 30 m, 700 °C oxidation treatment. ( b ) EXAFS Fourier transform plots showing (A) the state of the starting catalyst, and (B) the growth of Pd metal during CO oxidation. The catalyst was heated to 300 °C under CO oxidation and then re-oxidized at 700 °C, restoring the catalyst to its starting state (C). Full size image To explore the structural relationship between La and Pd on γ-alumina, a more detailed analysis of the EXAFS data obtained from the initial-state samples was performed. Examination of several lanthanum palladates reveals a common structural relationship between Pd and La in these compounds, involving square-planar Pd connected to La through two bridging oxygens. The compound La 2 PdO 4 was chosen to serve as an analogue, providing initial estimates of structural parameters ( Fig. 7a ). Integration of this structural relationship with the γ-alumina structure was achieved by placing the La atom into the four-fold hollow site provided by an Al 3+ vacancy [15] , and by replacing an adjacent penta-coordinated Al 3+ ion (ionic radius (VI octahedral) 0.53 Å) with a Pd 2+ ion (ionic radius (IV square planar) 0.64 Å) [25] ( Fig. 7b ). The resulting Pd environment, used in the fit to the EXAFS data, is shown in Fig. 7c . The apical oxygen, shown in Fig. 7c , was omitted from the fits, as inclusion of this oxygen was found to significantly reduce the precision of the fit variables. Although the EXAFS Fourier transform magnitude at values of R >2 Å is rather low, reasonable fits of the real and imaginary components ( Supplementary Fig. 9 ), and reasonable variable values and uncertainties were obtained ( Supplementary Table 6 ), demonstrating that the structure shown in Fig. 7b,c is a plausible representation of the structure of the atomically dispersed Pd on the alumina surface. 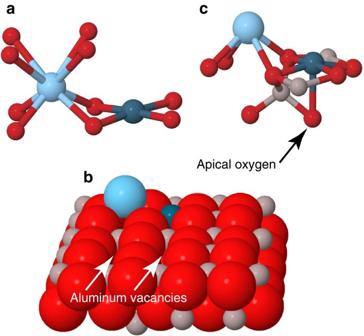Figure 7: Model for the La and Pd on the γ-alumina (100) surface. (a) La and Pd relationship in the La2PdO4structure. (b) Space-filling γ-alumina (100) surface model (spinel basis) with La and Pd. (c) Model for EXAFS fit, based onb. Atoms are: oxygen/red, aluminum/grey, palladium/dark blue and lanthanum/light blue. Figure 7: Model for the La and Pd on the γ-alumina (100) surface. ( a ) La and Pd relationship in the La 2 PdO 4 structure. ( b ) Space-filling γ-alumina (100) surface model (spinel basis) with La and Pd. ( c ) Model for EXAFS fit, based on b . Atoms are: oxygen/red, aluminum/grey, palladium/dark blue and lanthanum/light blue. Full size image DFT calculations To corroborate the experimental results, plane-wave DFT calculations have been performed using the Vienna ab initio simulation package [26] , [27] , [28] with the gradient-corrected PW91 exchange-correction functional [29] . Our model for Pd-doped γ-alumina involves the (001) surface of Al 2 O 3 (ref. 7 ; Supplementary Fig. 10 ) (four-fold symmetry) with Pd replacing a surface Al. The details of the DFT calculations and additional results, including the optimized surface structures ( Supplementary Fig. 11 ) can be found in the Supplementary Discussion. Supported single Pd atoms have been predicted [30] to diffuse easily across the Al 2 O 3 surfaces with diffusion barriers on the order of 0.3 eV, and are expected to nucleate [31] quickly to form larger clusters. However, when incorporated into the alumina lattice the Pd atom has both the binding energy and geometrical arrangement necessary to account for the experimental observations that show four-fold coordination with oxygen atoms. A comparison of the local density of states calculated for the Pd(111) surface with that calculated for Pd substituted into the alumina structure is shown in Supplementary Fig. 12 . A reaction mechanism is proposed based on the DFT calculations as displayed in Fig. 8 , where the energetics are also shown. In this putative mechanism, the catalytic cycle is initiated by the adsorption of CO onto the Pd, which then reacts with a lattice oxygen (O lat ) coordinated with Pd. After overcoming an activation barrier of 0.26 eV, an intermediate (INT1) was found with E r =−0.46 eV. At the transition state, the C–O bond length and the C–O lat distance are computed to be 1.16 and 1.82 Å, respectively. Several steps are needed to eventually produce CO 2 , which promptly desorbs removing O lat in the process. The second half of the catalytic cycle starts with the newly formed oxygen vacancy from the first step, in which Pd is now coordinated to three lattice oxygen atoms with distances of 2.15, 2.27 and 2.49 Å. The adsorption of an O 2 molecule (O 2 gas /O gas ) at the vacancy is highly exothermic, with its bond length elongated from 1.23 Å in the isolated molecule to 1.45 Å. This is followed by the adsorption of CO on Pd, which promptly reacts with the pre-adsorbed O 2 gas nearby. This step has an energy barrier of 0.27 eV and the exothermicity is found to be −3.66 eV. At the transition state, the C–O and the C–O gas bond lengths are calculated to be 1.16 and 1.94 Å, respectively. By releasing the CO 2 product, the Pd recovers its tetra-coordinated state on the γ-Al 2 O 3 (100) surface. Additional results from the DFT calculations, including geometry, energetics and charge analyses, can be found in the Supplementary Discussion. 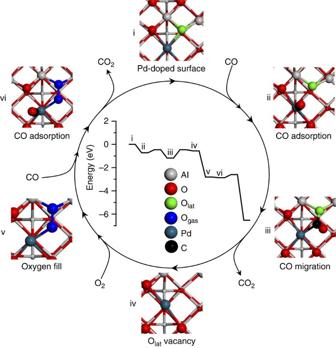Figure 8: Proposed reaction mechanism for CO oxidation on isolated Pd on the γ-alumina (100) surface. The initial state (i) consists of square planar Pd in Al vacancy defect followed by CO adsorption on Pd (ii). CO2is formed by removing an oxygen atom from the surface (iii), resulting in a vacancy (iv). Molecular oxygen is adsorbed in theOlatvacancy (v) and a second CO molecule is adsorbed (vi) and oxidized completing the catalytic cycle. Figure 8: Proposed reaction mechanism for CO oxidation on isolated Pd on the γ-alumina (100) surface. The initial state (i) consists of square planar Pd in Al vacancy defect followed by CO adsorption on Pd (ii). CO 2 is formed by removing an oxygen atom from the surface (iii), resulting in a vacancy (iv). Molecular oxygen is adsorbed in the O lat vacancy (v) and a second CO molecule is adsorbed (vi) and oxidized completing the catalytic cycle. Full size image The stabilization of atomically dispersed transition metals such as Au, Pt and Rh on reducible oxides such as TiO 2 , FeO x and CeO 2 has been reported recently [2] , [3] , [20] . These catalysts have been shown to be active for reactions such as CO oxidation, water gas shift and also for olefin hydrogenation. However, reports on the stabilization of precious metals on high surface alumina are very scarce [9] , [32] . The presence of atomically dispersed Pd on alumina was suggested based on XPS spectra in the early 80s. Hence, the present study is consistent with these previous observations that have demonstrated that the alumina surface has sites where isolated ionic forms of transition metals can be present. What has not been recognized in previous work is that atomically dispersed La 3+ may play an important role in stabilizing ionic forms of Pd 2+ on the alumina surface. We showed previously [18] , [33] that the presence of the La 3+ on the surface may also help in slowing rates of catalyst sintering and help nucleate sub-nanometre clusters of the metal that may be responsible for the enhanced reactivity seen on the La-alumina catalysts. As isolated single-atom species may not be stable during reaction, it is necessary for practical applications to develop methods to regenerate these species. We show in this work that high-temperature calcination in air helps to re-disperse the Pd and restore catalytic activity. The atomic dispersion of the Pd after high-temperature calcination was confirmed by XAS; we have also performed AC-STEM studies to verify this re-dispersion process. The energetics of re-dispersion of Pd suggests that sub-nanometre clusters of Pd may be easier to disperse through this route, while bulk PdO is very stable and may not be easily redispersed. A high-temperature calcination step (700 °C) seems to be most effective at restoring catalytic activity of the isolated Pd species, although 500 °C calcination was also found to partially restore the lost catalytic activity. It is possible that desorption of hydroxyl groups from the alumina surface facilitates the re-dispersion process (we see evidence for loss of water during calcination). It was shown recently that calcination of alumina to 700 °C creates a more active form of alumina [34] . As oxidation of Pd commences around 200 °C and is complete by 500 °C, the beneficial effect of higher-temperature calcination must be the rearrangements on the alumina surface that are perhaps similar to those described by Wischert et al . [34] The facile re-dispersion of single isolated Pd atoms makes this Pd/alumina system more suitable for industrial applications. DFT computations in the literature suggest that among the transition metals, Pd would probably be the most strongly bound to alumina [32] . This may explain why we are able to generate catalysts that are composed exclusively of isolated Pd species. Previous studies of single-atom catalysts of Au, Rh or Pt always reported the co-existence of the atomically dispersed and nanoparticle phases, making it difficult to derive specific reactivity for the single-atom species. In several studies, the authors leached out the nanoparticle phase (for example using cyanide), leaving behind the atomically dispersed species on the support. This step was not needed in our experiments due to the higher stability of the Pd on alumina, especially in the presence of La 3+ . The study of complex oxides has shown that cations of Pd, Au or Pt can be stabilized in these oxides [35] . A common feature in these mixed oxides is the presence of high oxidation state cations such as La 3+ . We therefore believe that the role of La 3+ on the alumina surface is similar to that in these mixed oxides. For oxidation reactions, the proposed mechanism involves the participation of oxygen atoms from the support. In the case of reducible oxides, it is expected that the removal of oxygen from the support is facile causing the cations in the support to change oxidation state when it is reduced. This is the case with CeO 2 or TiO 2 that are known to be easy to reduce. However, these reducible oxide supports are also susceptible to loss of surface area during high-temperature operation, and they tend to form strongly bound carbonates or other reaction products that can poison the catalyst. There have been very few reports of the reactivity of atomically dispersed Pd on non-reducible supports such as alumina [10] , [17] , [32] . The presence of atomically dispersed Pt has been demonstrated previously [9] , [10] , but these species show CO oxidation light-off temperature higher than that of Pt metal [36] . Our results show that the atomically dispersed Pd sites show exceptional activity at low temperatures where metallic Pd surface sites are not active because they are poisoned by strongly adsorbed CO. The ionic form of Pd is not poisoned by adsorbed CO, as it is bound less strongly, consistent with the positive order in CO oxidation kinetics. The weakly bound, reversible CO adsorption seems to be the key difference between Pd metal sites and isolated atomic species. Providing oxygen from the support makes it possible to complete the catalytic cycle with a lower activation barrier than on metallic Pd. The barrier calculated from the DFT calculations (0.27 eV) is similar to the apparent activation energy measured experimentally. Furthermore, as the oxygen comes from the support, it is therefore reasonable that the order of reaction with oxygen is near zero. As we explain in the Supplementary Discussion, doping of the ionic Pd in alumina (which is achieved only after high-temperature calcination) yields oxygen atoms that bridge the Al and Pd sites. These bridging oxygens, being different from those seen on stable alumina surfaces, can participate in the CO oxidation reaction. We therefore propose a reaction mechanism that differs from the conventional Langmuir Hinshelwood mechanism, which operates on metallic Pd surfaces. The Bader charge analysis presented in the Supplementary Discussion shows that we should not consider these active sites as being single-atom analogues of homogeneous catalysts, but rather they involve the participation of the extended alumina support surface. In summary, this work shows how atomically dispersed La 3+ ions may play a key role in helping to stabilize atomically dispersed ionic Pd on the alumina surface. Our XANES results show that atomically dispersed Pd 1+ is the active centre for CO oxidation, and that the catalytic behaviour of these species is very different from that of Pd metal. A novel catalytic mechanism is proposed to explain the unexpected reactivity for the isolated Pd species. The ability to atomically disperse transition metals on industrially relevant high-surface-area supports paves the way to develop more efficient use of expensive platinum group metals as catalysts. Electron microscopy AC HAADF images were collected at Oak Ridge National Laboratory—High Temperature Materials Laboratory, using a JEOL 2200FS electron microscope, equipped with a CEOS GmbH (Heidelburg, Germany) corrector on the probe-forming lenses. Images were obtained from a sample composed of La-alumina (4 wt% La 2 O 3 ; W. R. Grace (MI-386)), loaded with 2.5 wt% Pd. Images were also collected from the same support material, without Pd, for comparison with the images obtained from the Pd-loaded sample. Measurement of the electron backscatter intensity was performed by fitting two-dimensional Gaussian functions to the clusters of atoms seen in the images, using a MATLAB algorithm. Catalyst preparation For the alumina support, Dispal (boehmite) from Sasol was calcined at 650 °C for 10 h to make γ-alumina, and the Brunauer-Emmett-Teller (BET) surface area was determined to be 153 m 2 g −1 . The La-alumina support, containing 4 wt% La 2 O 3 , was obtained from W. R. Grace (MI-386), and has a BET surface area of 176 m 2 g −1 . The BET surface areas were measured on a Micromeritics Gemini 2360 instrument under liquid nitrogen at 77 K. Samples were prepared by dry impregnation of γ-alumina powders with a solution of palladium amine nitrate, diluted to the appropriate concentration to achieve 0.5 wt% Pd loading after three impregnations. Samples were dried at 110 °C after each impregnation, and finally calcined at 700 °C for 1 h in a box furnace in ambient air. The temperature was raised at a slow rate 2 °C min −1 to help generate the best dispersion of the Pd oxide phase. CO oxidation reactivity For CO oxidation reactivity measurements, 100 mg of sample was packed between quartz wool plugs inside a stainless steel reactor tube mounted in a high-temperature oven. The sample was pretreated as follows: 100 mg of sample was heated to 700 °C under O 2 /He for at least 30 min. Samples were cooled under oxidizing conditions to room temperature where the CO oxidation reaction mixture was introduced. The flow rates consisted of 0.8 ml min −1 O 2 , 0.7 ml min −1 CO and 70 ml min −1 He. The samples were then heated to 300°C at 2°C min −1 and cooled back down to room temperature in the reaction mixture, and a second, identical ramp was then performed. Reaction kinetics measurements were conducted after another 700 °C pretreatment, and then cooling the sample to 70 °C. The reactant mixtures were allowed to flow, and as the catalyst activity was lost over time, the reactant flow rates were varied by either increasing the O 2 flow rate while keeping CO flow constant or by an increase in CO flow rate with constant O 2 flow. Exit gas composition was measured using a Varian CP-4900 Micro-GC gas chromatograph, using a thermal conductivity detector (TCD) detector. X-ray absorption spectroscopy Operando XAS was performed at the Argonne National Laboratory Advanced Photon Source beam-line 10-ID-B. The samples (200 mg) were packed into 10 mm (I.D.) quartz NMR tubes, which were open at both ends, and were supported between two quartz wool plugs. The tubes were mounted vertically in a tube furnace and gas flow was from top to bottom through the packed sample bed. Gas flow rates were controlled using Sierra mass flow controllers. The exit gas composition was analysed using the same Varian CP-4900 Micro-GC gas chromatograph. After being loaded into the reactor tube, the samples were given an oxidizing pretreatment in flowing 1% O 2 /He at 50 ml min −1 , by ramping to 700 °C at 20 °C min −1 and holding for 30 min. The samples were then cooled to room temperature under flowing gas, and XAS data was collected, without intervening exposure to ambient air. The CO reaction mixture consisted of 0.7 ml min −1 CO, 0.8 ml min −1 O 2 , diluted in He with a total gas flow rate of 140 ml min −1 . This was achieved by mixing ~1% O 2 /He and ~1% CO/He using the mass flow controllers. The experimental procedure was to ramp the temperature with the CO flow turned off, stabilize the temperature, turn on the CO flow for 30–45 min, and finally turn the CO off and ramp to the next temperature. (Turning off the CO gas feed reduced the total flow by approximately one half.) Gas analysis and XAS collection were performed continuously during these changes in flow rates and temperatures. The XANES and EXAFS data were analysed using the Athena and Artemis software [37] , [38] . Palladium oxide and metal fractions were determined from linear combination fits of XANES Pd-oxide and metal end member standards. The XANES spectrum obtained from the initial, post-700 °C oxidation state of each catalyst was chosen as the palladium oxide standard. It was assumed that this spectrum represented atomically dispersed palladium in square-planar coordination with oxygen, and palladium oxide S 0 2 values were refined for the alumina and La-alumina samples using these spectra. Pd-foil reference spectra were chosen as the Pd metal standards. In the non-isosbestic cases (that is, when Pd-metal was present in La-alumina-supported catalyst), a third linear combination standard, representing Pd δ+ , was used. The metal-free sample with the smallest Pd-O coordination number (the final 80 °C CO-oxidation spectrum) was chosen to represent this end member. The EXAFS data was analysed using a two-phase, oxide/metal model. The phase fractions were fixed at the values obtained from the linear combination fits of the XANES data. The Pd-oxide Pd-O and Pd-metal Pd-Pd coordination numbers were refined for each spectrum with the Pd-oxide and Pd metal S 0 2 values fixed at those obtained from the Pd-oxide and metal standards. How to cite this article: Peterson, E. J. et al . Low-temperature carbon monoxide oxidation catalysed by regenerable atomically dispersed palladium on alumina. Nat. Commun. 5:4885 doi: 10.1038/ncomms5885 (2014).